Attenuation of nonsense-mediated mRNA decay facilitates the response to chemotherapeutics Nonsense-mediated mRNA decay (NMD) limits the production of aberrant mRNAs containing a premature termination codon and also controls the levels of endogenous transcripts. Here we show that when human cells are treated with clinically used chemotherapeutic compounds, NMD activity declines partly as a result of the proteolytic production of a dominant-interfering form of the key NMD factor UPF1. Production of cleaved UPF1 functions to upregulate genes involved in the response to apoptotic stresses. The biological consequence is the promotion of cell death. Combined exposure of cells to a small-molecule inhibitor of NMD, NMDI-1, and the chemotherapeutic doxorubicin leads to enhanced cell death, while inhibiting UPF1 cleavage protects cells from doxorubicin challenge. We propose a model to explain why the expression levels of genes producing mRNAs of diverse structure that encode proteins of diverse function are under the purview of NMD. An estimated approximately one-third of inherited diseases are the result of premature termination codon (PTC) acquisition [1] . Nonsense-mediated mRNA decay (NMD) is a conserved mRNA quality-control pathway deployed by cells to eliminate mRNAs containing a PTC. Because proteins produced by PTC-containing mRNAs may have deleterious consequences, selection and destruction of these mRNAs by NMD maintains cellular homeostasis. Less well understood, but equally important, is the role of NMD in maintaining and regulating the levels of endogenous, non-mutated transcripts [2] , [3] , [4] , [5] , [6] , [7] . These transcripts are of heterogeneous structure and encode proteins of heterogeneous function, yet they have the unifying feature that disrupting NMD elicits their upregulation [2] , [3] , [4] , [5] , [6] , [7] . How NMD-mediated changes in the levels of these transcripts are integrated into cellular physiology is unclear for all but a few situations. During muscle cell differentiation in humans and rodents, NMD efficiency is downregulated, while the efficiency of a competing pathway, Staufen-mediated mRNA decay, is upregulated [8] , [9] . These changes tailor the mRNA pool to favour the expression of promyogenic factors [8] , [9] . During hypoxia, the efficiency of NMD is inhibited, promoting tumorigenesis [10] . Additional stresses that cause eukaryotic initiation factor 2α phosphorylation can also inhibit NMD, but how this is achieved remains unclear [11] , [12] . A better-understood example involves the developmental programme underlying the differentiation of neural stem cells (NSCs), during which a neural-specific microRNA, miR-128, is expressed. miR-128 targets the core NMD factor UPF1, downregulating the efficiency of NMD and upregulating the abundance of transcripts involved in post-mitotic NSC differentiation [5] , [13] . Destruction of NMD targets is the result of incompletely understood mRNP rearrangements [1] , [14] . Target selection is strictly dependent on translation and the result of one of at least five classes of cis -residing transcript features: (i) an upstream open reading frame in the 5′ untranslated region (UTR) where the stop codon of the upstream open reading frame is a PTC relative to the main ORF and also resides ≥50–55 nts upstream of an exon-exon junction so that the exon-junction complex (EJC) of proteins deposited upstream of the exon-exon junction fails to be removed by translating ribosomes; (ii) alternative pre-mRNA splicing that generates a shift in the translational reading frame and a PTC ≥ 50–55 nts upstream of an exon-exon junction or generates an exon-exon junction ≥ 50–55 nts downstream of the normal termination codon; (iii) abnormally long 3′ UTRs; (iv) a UGA codon within specialized selenoprotein mRNAs that encodes selenocysteine with less than 100% efficiency, resulting in PTC-triggered NMD; or (v) a normal stop codon ≥50–55 nts upstream of a splicing generated exon–exon junction [1] . In a model of EJC-mediated NMD, the terminating ribosome nucleates a complex termed ‘SURF’, which is composed of the protein kinase SMG1, the key NMD factor UPF1, and eukaryotic release factors 1 and 3, on the mRNA to be degraded [15] . The EJC is decorated with NMD factors UPF3 or UPF3X and UPF2 that, on UPF1 binding, promote the ATP-dependent RNA helicase activity of UPF1 (refs 16 , 17 ). The defining feature of an mRNA that is destined for destruction is the presence of phosphorylated UPF1 (p-UPF1) [7] , [15] , [18] , [19] . SMG1 phosphorylates human UPF1 in both its amino (N)- and carboxyl (C)-terminal tails [18] . p-UPF1 then recruits SMG6 RNA endonuclease [20] , [21] , [22] , and/or SMG5–SMG7 or SMG5–PNRC2 complexes, the latter two of which further recruit RNA deadenylating and decapping activities that precede exonucleolytic activities [23] , [24] , [25] , [26] , [27] . Administration of small-molecule anticancer drugs is a mainstay of cancer treatment. Among the drugs used are topoisomerase inhibitors, such as doxorubicin, which cause double-stranded DNA breaks. DNA damage activates the p53 tumour suppressor pathway, an early consequence of which is the inhibition of cell division [28] . In cases of severe DNA damage, regulated cell death or apoptosis ensues [28] . How cells that are exposed to apoptotic insults deal with apoptotic stresses has only been recently studied [29] . Clearly there is dynamic resculpting of the proteome and the transcriptome: a transcriptional response (for example, by the p53 network) precedes the loss of cellular metabolism. Concomitant with a decrease in cellular viability is a global decrease in mRNA levels [30] , [31] . Superimposed on these changes are proteolytic events, carried out by caspase enzymes that actively promote apoptosis and dismantle the cell [32] , [33] . Here we examine how NMD is integrated into the network of processes that define the apoptotic response. We find that NMD is inhibited during apoptosis, in part, by the proteolytic production of a dominant-interfering form of UPF1. Inhibiting UPF1 cleavage protects cells from the effects of doxorubicin. Conversely, decreasing the efficiency of NMD using a small-molecule inhibitor sensitizes cells to doxorubicin. We propose that the efficiency of NMD can be tuned by extracellular stimuli, and one purpose for the NMD-mediated control of endogenous gene expression is to assist in the establishment of a particular state by tailoring the mRNA milieu to one that can respond to potentially diverse stimuli. NMD activity is blunted during doxorubicin treatment We examined the stability of a panel of known NMD target mRNAs [34] in human MCF7 breast cancer cells during doxorubicin treatment. Pretreatment with doxorubicin (5 μM) resulted in significant increases in the half-lives of PANK2, TSTD2 and NAT9 mRNAs but not β-actin mRNA after actinomycin D-mediated transcriptional arrest ( Fig. 1a ), indicating a decline in NMD activity. To support this, we measured the level of each mRNA relative to the level of the pre-mRNA from which it derives as a function of time after doxorubicin treatment to control for transcriptional effects. An increase in the mRNA/pre-mRNA ratio (a metric used to distinguish a subset of direct NMD targets from those that are not in UPF1-ablated HeLa cells [35] , [36] ) may not reliably distinguish NMD targets from those that are not during doxorubicin treatment, because global transcriptional shut-down may inflate this number. However, a decrease in this ratio would rule out the possibility that NMD activity is blunted. Consistent with our half-life data, the mRNA/pre-mRNA ratio, as assessed using reverse transcription (RT)–quantitative PCR (qPCR), increases for all three transcripts (none of which is known to be stress regulated), in response to doxorubicin ( Supplementary Fig. 1a ). The mRNA/pre-mRNA ratios for three additional known NMD-targeted transcripts [34] , [35] , [36] , [37] , [38] , CDKN1A, GADD45α and GADD45β, were also significantly increased by 5 h of doxorubicin treatment. As in HeLa cells, the ratio of CDKN1A, GADD45α and GADD45β mRNAs to their corresponding pre-mRNAs is elevated on UPF1 depletion in MCF7 cells, indicating that these mRNAs are indeed NMD targets in MCF7 cells ( Supplementary Fig. 1b ). Decreases in pre-mRNA levels cannot account for the increased mRNA/pre-mRNA ratio since, even in the most extreme example (CDKN1A RNA), at 5 h the mRNA/pre-mRNA ratio increased ~5.7-fold relative to 0 h, while the pre-mRNA level decreased only ~3.2-fold. 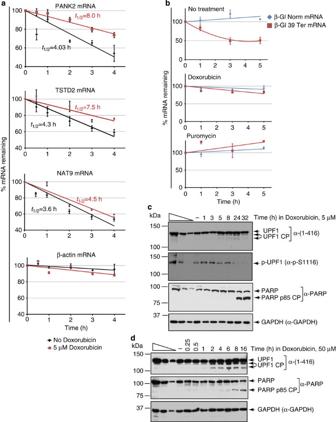Figure 1: NMD is inhibited during doxorubicin treatment. (a) mRNA decay assays in MCF7 cells. MCF7 cells either were (red) or were not (black) pretreated with 5 μM doxorubicin for 1 h before addition of 3 μg ml−1actinomycin D to halt transcription. Cells were collected at the indicated times after actinomycin D addition. Levels of the indicated NMD-targeted mRNAs were assessed by RT–qPCR, normalized to 18S rRNA levels and displayed as a percentage of the levels att=0 h. Error bars=s.e.m.,n=4 independent biological quadruplicates. (b) Human β-Gl mRNA half-life studies in HeLa Tet-off cells. HeLa Tet-off cells were transfected with plasmids encoding human β-Gl Norm mRNA and MUP mRNA or β-Gl Ter mRNA and MUP mRNA. β-Gl Norm and β-Gl 39 Ter mRNA transcription occurs under the agency of the non-stress-responsive Tet-off promoter. Cells were either pretreated with nothing (top), 50 μM doxorubicin for 1 h (middle) or 50 μg ml−1puromycin for 3 h (bottom) before transcriptional shut-off with 2 μg ml−1doxycycline. Cell aliquots were removed at the indicated ‘chase’ time points, and RT–qPCR was used to assess the remaining levels of β-Gl Norm and β-Gl Ter mRNAs, each after normalization to MUP mRNA. (c) Western blots of lysates of MCF7 cells from (Supplementary Fig. 1a) (blots derive from and are representative of the three biological replicates inSupplementary Fig. 1athat had been exposed to doxorubicin (5 μM) for the indicated times. GAPDH levels serve as loading controls. Threefold serial dilutions (wedge) reveal the dynamic range of analysis. α, anti; 1-416, UPF1 amino acids; CP, cleavage product. (d) As inc, but cells were exposed to a 10-fold higher concentration of doxorubicin and analysed at earlier time points. Representative of two biological replicates. Figure 1: NMD is inhibited during doxorubicin treatment. ( a ) mRNA decay assays in MCF7 cells. MCF7 cells either were (red) or were not (black) pretreated with 5 μM doxorubicin for 1 h before addition of 3 μg ml −1 actinomycin D to halt transcription. Cells were collected at the indicated times after actinomycin D addition. Levels of the indicated NMD-targeted mRNAs were assessed by RT–qPCR, normalized to 18S rRNA levels and displayed as a percentage of the levels at t =0 h. Error bars=s.e.m., n =4 independent biological quadruplicates. ( b ) Human β-Gl mRNA half-life studies in HeLa Tet-off cells. HeLa Tet-off cells were transfected with plasmids encoding human β-Gl Norm mRNA and MUP mRNA or β-Gl Ter mRNA and MUP mRNA. β-Gl Norm and β-Gl 39 Ter mRNA transcription occurs under the agency of the non-stress-responsive Tet-off promoter. Cells were either pretreated with nothing (top), 50 μM doxorubicin for 1 h (middle) or 50 μg ml −1 puromycin for 3 h (bottom) before transcriptional shut-off with 2 μg ml −1 doxycycline. Cell aliquots were removed at the indicated ‘chase’ time points, and RT–qPCR was used to assess the remaining levels of β-Gl Norm and β-Gl Ter mRNAs, each after normalization to MUP mRNA. ( c ) Western blots of lysates of MCF7 cells from ( Supplementary Fig. 1a ) (blots derive from and are representative of the three biological replicates in Supplementary Fig. 1a that had been exposed to doxorubicin (5 μM) for the indicated times. GAPDH levels serve as loading controls. Threefold serial dilutions (wedge) reveal the dynamic range of analysis. α, anti; 1-416, UPF1 amino acids; CP, cleavage product. ( d ) As in c , but cells were exposed to a 10-fold higher concentration of doxorubicin and analysed at earlier time points. Representative of two biological replicates. Full size image To further corroborate the inhibition of NMD during doxorubicin treatment, we transfected MCF7 cells with the previously described β-globin (β-Gl) NMD reporter plasmids [39] encoding either β-Gl Norm transcripts that lack a PTC, or β-Gl Ter transcripts that harbour a PTC at position 39. Cells were co-transfected with a plasmid encoding the mouse urinary protein (MUP) transcript to control for variations in transfection efficiency and RNA recovery and, 24 h later, were exposed to doxorubicin (5 μM). After 5 h of doxorubicin treatment, the level of β-Gl Ter mRNA increased from ~65 to ~85% the level of β-Gl Norm mRNA. These measurements occur on the backdrop of global RNA degradation at later time points [29] , [30] , accounting for why the normalized ratio of β-Gl Ter mRNA to β-Gl Norm mRNA is not elevated at later time points. We performed additional mRNA decay assays using a previously described human cervical carcinoma HeLa cell Tet-off cell system [40] to halt the synthesis of human β-Gl Norm mRNA or β-Gl Ter mRNA and subsequently measured the remaining levels of each mRNA relative to the level of MUP mRNA after doxycycline addition. We used this system because the Tet-off promoter that controls the production of β-Gl Norm mRNA or β-Gl Ter mRNA is not stress responsive and HeLa cells, like MCF7 cells, are devoid of erythroid cell-specific β-Gl mRNA. Without doxorubicin, the level of β-Gl Ter mRNA declined to ~50% of its starting level by ~180 min of doxycycline addition, in agreement with reported values [40] , while the level of β-Gl Norm mRNA did not decrease during this time ( Fig. 1b ; top). In contrast, pretreatment of cells with doxorubicin for 1 h before doxycycline addition eliminated the selective decay of β-Gl Ter mRNA; the half-lives of both β-Gl Norm mRNA and β-Gl Ter mRNA exceeded the chase period ( Fig. 1b ; middle). Doxorubicin treatment mirrored the effect of the translational inhibitor puromycin, which is known to inhibit NMD ( Fig. 1b ; bottom). From all results, we conclude that NMD activity is attenuated during doxorubicin treatment. We next examined biochemical changes to the key NMD factor, UPF1, that correlate with doxorubicin treatment ( Fig. 1c ). We exposed MCF7 cells to doxorubicin (5 μM) for varying amounts of time and analysed cell lysates using western blotting and an in-house generated polyclonal rabbit serum raised against the N-terminal 416 amino acids of human UPF1. To eliminate post-lysis proteolysis, lysates were generated in the presence of a protease inhibitor cocktail supplemented with N -ethylmaleimide at levels (50 μg ml −1 ) known to alkylate the most active viral cysteine proteases. In addition to full-length UPF1, two additional bands of greater mobility were resolved by 5 h of doxorubicin treatment ( Fig. 1c ). Phosphorylation of UPF1 at both its N- and C termini is a key feature that differentiates UPF1-bound NMD targets destined for degradation from those that are not [7] , [15] , [41] , [42] . Western blotting using a monoclonal antibody recognizing phosphorylated S1116 revealed that UPF1 phosphorylation levels diminish by 5 h. Both of these changes to UPF1 preceded maximal cleavage of poly (ADP-ribose) polymerase (PARP), a well-characterized biochemical marker for apoptosis. Increasing doxorubicin concentrations 10-fold (50 μM) to accelerate apoptotic progression generated higher-mobility UPF1 species by 2 h, that is, well before the production of the PARP cleavage product (CP) at 8 h ( Fig. 1d ). Thus, the generation of faster-migrating UPF1 species, which we characterize as cleavage products (CPs) (see below), and the reduction of UPF1 phosphorylation occur early during apoptotic progression (see below). Multiple apoptotic insults cause UPF1 hydrolysis We characterized the upper UPF1 CP because we observed that it was consistently generated by an array of treatments in many cell lines (see below). We verified that this band derives from cellular UPF1 rather than a protein that fortuitously cross-reacts with our polyclonal anti-UPF1 serum by using short interfering RNA (siRNA) to reduce the level of UPF1 in HeLa cells to <10% of normal and subsequently exposing cells to cycloheximide (CHX) to induce apoptosis ( Fig. 2a ). In addition to halting protein synthesis, CHX causes apoptosis via incompletely understood mechanisms [43] . siRNA treatment reduced the levels of both full-length UPF1 and the UPF1 CP. Because new protein synthesis is halted by CHX, the UPF1 CP is unlikely to be a UPF1 isoform explained by the hypothetical possibility that alternative splicing of UPF1 pre-mRNA is induced during apoptosis. 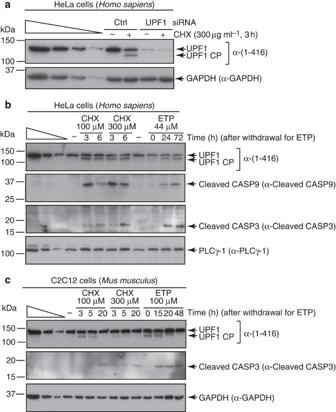Figure 2: UPF1 CP production is an early and conserved event. (a) Western blots of lysates of HeLa cells (Homo sapiens) transfected with 100 nM of either control (Ctrl) siRNA or UPF1 siRNA and, 48 h later, exposed to CHX (300 μg ml−1) for 3 h. (b) Western blots of lysates of HeLa cells (Homo sapiens) exposed to CHX (100 or 300 μg ml−1) for either 3 or 5 h, or to ETP (44 μM) for 6 h, incubated in fresh medium and withdrawn from ETP at the indicated times. (c) Essentially as inbexcept C2C12 myoblasts (Mus musculus) were analysed. CHX concentrations were 100 or 300 μg ml−1, and a 5 h pulse of ETP was used at 100 μM. Note that at least two apoptotic inducers were used for each cell line, and at least two cell lines were tested with each apoptotic inducer. Figure 2: UPF1 CP production is an early and conserved event. ( a ) Western blots of lysates of HeLa cells ( Homo sapiens ) transfected with 100 nM of either control (Ctrl) siRNA or UPF1 siRNA and, 48 h later, exposed to CHX (300 μg ml −1 ) for 3 h. ( b ) Western blots of lysates of HeLa cells ( Homo sapiens ) exposed to CHX (100 or 300 μg ml −1 ) for either 3 or 5 h, or to ETP (44 μM) for 6 h, incubated in fresh medium and withdrawn from ETP at the indicated times. ( c ) Essentially as in b except C2C12 myoblasts ( Mus musculus ) were analysed. CHX concentrations were 100 or 300 μg ml −1 , and a 5 h pulse of ETP was used at 100 μM. Note that at least two apoptotic inducers were used for each cell line, and at least two cell lines were tested with each apoptotic inducer. Full size image Cleavage of proteins by caspases, a class of cysteine proteases, during apoptosis is a common event [32] , [33] . ‘Bystander’ cuts to proteins fortuitously encoding a caspase cleavage site may occur during apoptosis, but cleavage early during apoptotic progression and cleavage conservation across species indicate functional relevance [33] . To examine the timing of UPF1 CP generation, we treated HeLa cells with the clinically used topoisomerase inhibitor etoposide (ETP). ETP induced generation of a UPF1 CP before the full induction of cleaved initiator caspase 9 (CASP9) and cleaved executioner CASP3 ( Fig. 2b ). Generation of the UPF1 CP before full CASP9 and CASP3 cleavage is recapitulated in human embryonic kidney (HEK)293T cells during CHX treatment ( Supplementary Fig. 2a ). We examined the effects of other apoptotic inducers on UPF1 CP generation. Treatment of HEK293T cells with staurosporine also yielded two UPF1 CPs, before full cleavage of CASP9 and CASP3 ( Supplementary Fig. 2b ). Exposure of the human Daudi B-lymphoblast cell line to either tumour necrosis factor-α or doxorubicin led to the generation of the UPF1 CP before maximal PARP cleavage ( Supplementary Fig. 2c ). Staurosporine-challenged Jurkat T cells also yielded a UPF1 CP before maximal cleavage of CASP3 or PARP ( Supplementary Fig. 2d ). To probe whether generation of the UPF1 CP is evolutionarily conserved, we exposed mouse C2C12 myoblasts to CHX or ETP, both of which generated a UPF1 CP before maximal CASP3 cleavage ( Fig. 2c ). Exposure of canine (MDCK), bovine (MDBK) and Chinese hamster (CHO) cells to staurosporine led to UPF1 CP production ( Supplementary Fig. 2e–g ). Likewise, exposure of African Green monkey (COS-7) cells to staurosporine or doxorubicin yielded a UPF1 CP ( Supplementary Fig. 2h ). UPF1 CP levels varied drastically across cell lines, likely for three reasons: (i) in non-human cells, we cannot assess how efficiently our treatments elicited apoptosis because antibodies to human PARP, cleaved human CASP9 and cleaved human CASP3 do not cross-react; (ii) our anti-UPF1 antiserum was raised against the first 416 amino acids of human UPF1 and may exhibit reduced cross-reactivity to non-human UPF1 CP; and (iii) as a result of cleavage at the N terminus (see below), the human UPF1 CP exhibits less than one-third the immunoreactivity of full-length human UPF1 with our UPF1 antiserum. Notwithstanding this, UPF1 CP generation is an early event that is evolutionarily conserved, indicating that UPF1 cleavage may play a role in the cellular response to apoptotic induction. Mapping UPF1 hydrolysis To probe whether caspases are involved in UPF1 CP generation, we preincubated HEK293T cells with a panel of caspase inhibitors followed by exposure to CHX ( Fig. 3a ). Cells treated with each caspase inhibitor showed drastically reduced UPF1 CP levels, with Z-DEVD-fmk and Z-VAD-fmk lowering the level of UPF1 CP to nearly undetectable. Thus, caspases, and/or alternative proteases [44] activated downstream of caspases, are involved in UPF1 CP production. We exposed a HeLa cell line stably expressing N-terminally tagged FLAG-UPF1 (ref. 45 ) to CHX. While anti-FLAG immunoblots failed to reveal any UPF1 CP even after long exposure, anti-UPF1 immunoblots using antiserum raised against amino acids 1–416 ( Fig. 3b ) yielded detectible UPF1 CP ( Fig. 3c ), indicating that cleavage occurs within the first 416 amino acids of UPF1 so as to eliminate the FLAG epitope but preserve partial immunoreactivity with our UPF1 antiserum. 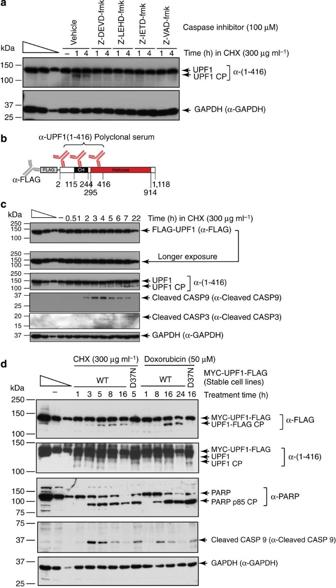Figure 3: UPF1 CP is produced by hydrolysis at aspartic acid 37. (a) Western blots of lysates of HEK293T cells preincubated with the indicated peptide-based fluoromethylketone caspase inhibitor for 4 h, before addition of CHX (300 μg ml−1) for the indicated times. (b) Diagram of N-terminally FLAG-tagged human UPF1, showing its reactivity with anti(α)-UPF1(1–416). CH, cysteine+histidine-rich region. (c) Western blots of lysates of HeLa cells stably expressing an N-terminally FLAG-tagged UPF1 and incubated with CHX for the indicated times. (d) Western blots of lysates of HeLa cells retrovirally transduced at a multiplicity of infection <0.1 with either MYC-UPF1-FLAG WT or MYC-UPF1-FLAG D37N (and thus G418 resistant) and exposed to CHX (300 μg ml−1) or doxorubicin (50 μM) in the absence of G418. Representative of two independent experiments. Figure 3: UPF1 CP is produced by hydrolysis at aspartic acid 37. ( a ) Western blots of lysates of HEK293T cells preincubated with the indicated peptide-based fluoromethylketone caspase inhibitor for 4 h, before addition of CHX (300 μg ml −1 ) for the indicated times. ( b ) Diagram of N-terminally FLAG-tagged human UPF1, showing its reactivity with anti(α)-UPF1(1–416). CH, cysteine+histidine-rich region. ( c ) Western blots of lysates of HeLa cells stably expressing an N-terminally FLAG-tagged UPF1 and incubated with CHX for the indicated times. ( d ) Western blots of lysates of HeLa cells retrovirally transduced at a multiplicity of infection <0.1 with either MYC-UPF1-FLAG WT or MYC-UPF1-FLAG D37N (and thus G418 resistant) and exposed to CHX (300 μg ml −1 ) or doxorubicin (50 μM) in the absence of G418. Representative of two independent experiments. Full size image Inventories of in vivo apoptotic cleavage events indicate that cleavage specificity in living cells is determined chiefly by an aspartic acid residue at the P1 position; P4–P2 residues contribute far less to specificity in cells than is indicated by in vitro -derived peptide-based substrate profiles [32] , [33] . Accordingly, we focused our attention solely on aspartic acid (D) residues in human UPF1 and interrogated residues D27, D37 and D75 near the UPF1 N terminus by mutating each to asparagine (N). Full-length wild-type (WT) UPF1 and, separately, each variant was expressed bearing an N-terminal MYC-tag and a C-terminal FLAG-tag in HeLa cells at a level equal to endogenous UPF1, and cells were subsequently challenged with CHX. For UPF1 WT, UPF1 D27N and UPF1 D75N, the UPF1 CP was generated at approximately one-third the level of uncleaved UPF1, as judged using an anti-FLAG immunoblot ( Supplementary Fig. 3a ). Both the UPF1 CP and uncleaved UPF1 retained the C-terminal FLAG tag, allowing unambiguous assessment of the ratio of UPF1 CP to full-length UPF1. UPF1 D37N yielded no UPF1 CP, indicating that the amide bond after D37 is the site of hydrolysis (that is, D37 is the P1 residue). We generated HeLa cells stably expressing one copy of retrovirally introduced MYC-UPF1-FLAG WT or MYC-UPF1-FLAG D37N transgene. Each protein was expressed at ~2.7-fold the level of endogenous UPF1 ( Fig. 3d ). In these cell lines, the D37N mutation abolished UPF1 CP generation in response to CHX and doxorubicin ( Fig. 3d ). MCF7 cells stably transduced with MYC-UPF1-FLAG WT also generated the UPF1 CP at approximately one-third the level of uncleaved UPF1 in response to doxorubicin, and the UPF1 CP matched the molecular weight of a UPF1 fragment encompassing residues 38–1118 ( Supplementary Fig. 3b ). We cannot detect the N-terminal 37 amino-acid fragment released on cleavage, likely either for technical reasons or because this fragment is unstable. Having established that one cleavage event occurs after position 37, we examined the conservation of surrounding amino acids by aligning UPF1 sequences from multiple species using ClustalX ( Supplementary Fig. 3c ). The putative consensus cleavage site EFTD is completely conserved in human, bovine, mouse and Xenopus laevis UPF1—it deviates in chicken UPF1 at a single amino acid (where D is G)—and harbours T at the P2 residue, consistent with the high frequency of S and T residues at P4, P3 and P2 residues in cellular apoptotic protein cleavage sites [32] . Previously confirmed caspase substrates also bear similar cleavage sites: protein kinase C ζ is cleaved after EETD [46] , and the NF-kB p65/RelA subunit is cleaved after VFTD [47] . We characterized which caspase(s) are sufficient to cleave UPF1 in vitro by treating immunoprecipitated samples of full-length MYC-UPF1-FLAG WT or the non-cleavable MYC-UPF1-FLAG D37N variant with recombinant caspases ( Supplementary Fig. 3d ). CASP3 and CASP7 cleaved MYC-UPF1-FLAG WT but not MYC-UPF1-FLAG D37N into a fragment with the same molecular weight as a Δ37-UPF1-FLAG variant lacking the N-terminal MYC-tag and first 37 residues of MYC-UPF1-FLAG WT (recapitulating the mapped UPF1 CP). This is consistent with our observation that Z-DEVD-fmk and Z-VAD-fmk blunt UPF1 CP production ( Fig. 3a ). UPF1 CP is not functional in NMD What might cleavage at D37 in human UPF1 accomplish? Both serine 10 (S10) and threonine 28 (T28) are phosphorylated by the NMD-associated kinase SMG1 (ref. 18 ), and phosphorylation is critical for NMD [7] , [18] , [19] , [41] , [42] . Cleavage would cause a loss of these phosphorylation sites and, indeed, experimental truncation of the first 35 amino acids in Arabadopsis thaliana UPF1 (causing loss of three phosphorylation sites) eliminates its NMD activity and causes it to act dominant negatively [48] . A previously described deletion of the N-terminal 63 amino acids of human UPF1 (dNT) causes loss of NMD activity and dominant-negative behaviour, as does mutation of the threonine 28 phosphorylation site to alanine [15] , [49] . We assayed the NMD activity of exogenously expressed UPF1 proteins without endogenous UPF1. We depleted endogenous UPF1 levels in HEK293T cells to <10% of normal using siRNA and subsequently transiently introduced one of several siRNA-resistant UPF1 expression vectors: MYC-UPF1-FLAG WT; MYC-UPF1-FLAG D37N; Δ37-UPF1-FLAG; MYC-UPF1-FLAG TEV (described later); MYC-UPF1 dNT [15] ; or MYC-UPF1 R843C, which abolishes UPF1 helicase activity [50] . Transfections included either a ‘Norm’ or a ‘Ter’ plasmid set to assess NMD activity. The ‘Norm’ set consists of the β-Gl Norm reporter plasmid, the MUP reference plasmid, and a T-cell receptor (TCR)β-based reporter plasmid. This TCRβ-based reporter plasmid contains a bidirectional promoter driving synthesis of an HA-Cerulean fluorescent protein and, in the opposite orientation, a 3 × FLAG-mCherry fluorescent protein whose transcript contains a 3′ UTR composed of a TCRβ minigene lacking introns (Δ JC intron) [51] ( Fig. 4a ). The ‘Ter’ plasmid set contains the β-Gl Ter reporter plasmid, the MUP reference plasmid and a TCRβ reporter plasmid bearing (+) the JC intron >55 nt downstream of the mCherry termination codon [51] rendering the mCherry transcript an EJC-mediated NMD substrate ( Fig. 4a ). Each variant was expressed at a level equivalent to endogenous UPF1 as assessed by comparing anti-UPF1, anti-MYC and anti-FLAG immunoblots ( Fig. 4b ). 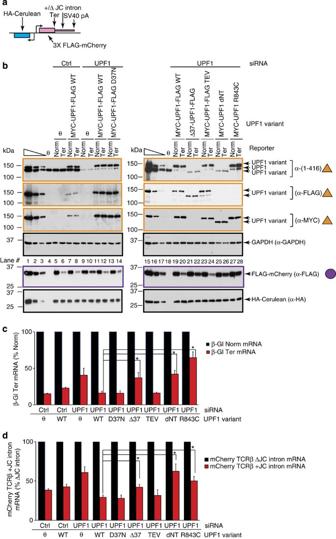Figure 4: UPF1 CP is not functional in NMD. (a) Schematic of TCRβ reporter plasmids. Bidirectional (two minimal cytomegalovirus) promoters (horizontal arrows) drive expression of HA-Cerulean protein (whose transcript is not an NMD target) and 3 × FLAG-mCherry protein. The TCRβ JC intron either does (+) or does not (Δ) reside >55 nt downstream of the 3 × -FLAG-mCherry termination codon (Ter), so that +JC intron transcripts are NMD targets, whereas ΔJC intron transcripts are not. pA, polyadenylation signal. (b) Western blots of lysates of HEK293T cells transfected with either control (Ctrl) siRNA or UPF1 siRNA (100 nM) and, 24 h later, with (i) the MUP reference plasmid, (ii) either the β-Gl Norm reporter plasmid plus the TCRβ reporter plasmid lacking the JC intron (ΔJC intron) or the β-Gl Ter reporter plasmid plus the TCRβ reporter plasmid containing the JC intron (+JC intron) and (iii) one of the following UPF1 variants: MYC-UPF1-FLAG WT (lanes 7,8,11,12,19,20); MYC-UPF1-FLAG D37N (lanes 13,14); Δ37-UPF1-FLAG (lanes 21,22); MYC-UPF1-FLAG TEV (lanes 23,24); MYC-UPF1 dNT (lanes 25,26); or MYC-UPF1 R843C (lanes 27,28). The level of each UPF1 variant was normalized to the level of GAPDH (orange triangles), while the level of 3 × FLAG-mCherry was normalized to the level of HA-Cerulean (purple circle). Blots derive from (and are representative of) the triplicate samples analysed inc. (c) RT–qPCR of RNA from samples analysed inbwhere β-Gl mRNA levels were normalized to the level of MUP mRNA, and the normalized level of β-Gl Norm mRNA in the presence of each UPF1 variant is defined as 100%. (d) RT–qPCR of RNA from samples analysed inbwhere 3 × FLAG-mCherry-TCRβ mRNA levels were normalized to the level of HA-Cerulean mRNA and the normalized level of 3 × FLAG-mCherry-TCRβ ΔJC intron mRNA in the presence of each UPF1 variant is defined as 100%. Error bars=s.e.m., *=P<0.05 relative to the UPF1 siRNA+MYC-UPF1-FLAG WT sample using the Student’st-test.n=3 independent biological replicates. Figure 4: UPF1 CP is not functional in NMD. ( a ) Schematic of TCRβ reporter plasmids. Bidirectional (two minimal cytomegalovirus) promoters (horizontal arrows) drive expression of HA-Cerulean protein (whose transcript is not an NMD target) and 3 × FLAG-mCherry protein. The TCRβ JC intron either does (+) or does not (Δ) reside >55 nt downstream of the 3 × -FLAG-mCherry termination codon (Ter), so that +JC intron transcripts are NMD targets, whereas ΔJC intron transcripts are not. pA, polyadenylation signal. ( b ) Western blots of lysates of HEK293T cells transfected with either control (Ctrl) siRNA or UPF1 siRNA (100 nM) and, 24 h later, with (i) the MUP reference plasmid, (ii) either the β-Gl Norm reporter plasmid plus the TCRβ reporter plasmid lacking the JC intron (ΔJC intron) or the β-Gl Ter reporter plasmid plus the TCRβ reporter plasmid containing the JC intron (+JC intron) and (iii) one of the following UPF1 variants: MYC-UPF1-FLAG WT (lanes 7,8,11,12,19,20); MYC-UPF1-FLAG D37N (lanes 13,14); Δ37-UPF1-FLAG (lanes 21,22); MYC-UPF1-FLAG TEV (lanes 23,24); MYC-UPF1 dNT (lanes 25,26); or MYC-UPF1 R843C (lanes 27,28). The level of each UPF1 variant was normalized to the level of GAPDH (orange triangles), while the level of 3 × FLAG-mCherry was normalized to the level of HA-Cerulean (purple circle). Blots derive from (and are representative of) the triplicate samples analysed in c . ( c ) RT–qPCR of RNA from samples analysed in b where β-Gl mRNA levels were normalized to the level of MUP mRNA, and the normalized level of β-Gl Norm mRNA in the presence of each UPF1 variant is defined as 100%. ( d ) RT–qPCR of RNA from samples analysed in b where 3 × FLAG-mCherry-TCRβ mRNA levels were normalized to the level of HA-Cerulean mRNA and the normalized level of 3 × FLAG-mCherry-TCRβ ΔJC intron mRNA in the presence of each UPF1 variant is defined as 100%. Error bars=s.e.m., *= P <0.05 relative to the UPF1 siRNA+MYC-UPF1-FLAG WT sample using the Student’s t -test. n =3 independent biological replicates. Full size image Comparing the levels of Δ37-UPF1-FLAG and MYC-UPF1 dNT with the level of MYC-UPF1-FLAG WT in immunoblots using the UPF1 a.a. 1–416, antiserum revealed a greater than threefold loss in immunoreactivity despite expression at equivalent levels (as assessed using anti-FLAG and anti-MYC immunoblots; Fig. 4b ). Comparing the level of β-Gl Ter mRNA with the level of β-Gl Norm mRNA revealed that Δ37-UPF1-FLAG is unable to promote NMD whereas MYC-UPF1-FLAG WT, MYC-UPF1-FLAG D37N and MYC-UPF1-FLAG TEV can: the β-Gl Ter mRNA level was ~2.4-fold higher in Δ37-UPF1-FLAG transfectants than in MYC-UPF1-FLAG WT transfectants ( Fig. 4c ). MYC-UPF1 dNT and MYC-UPF1 R843C were non-functional, yielding β-Gl Ter mRNA levels ~2.6- and ~4-fold higher than in MYC-UPF1-FLAG WT transfectants. These results were confirmed with the mCherry-TCRβ reporters ( Fig. 4d ). The anti-FLAG immunoblot of 3 × FLAG-mCherry protein (normalized to HA-Cerulean protein, whose level is unaffected by changes in NMD) revealed that the NMD substrate produces approximately twofold more protein in cells expressing non-functional Δ37-UPF1-FLAG, MYC-UPF1 dNT or MYC-UPF1 R843C relative to cells expressing MYC-UPF1-FLAG WT ( Fig. 4b ). Thus, UPF1 CP fails to support NMD. UPF1 CP is a dominant-interfering protein Could the UPF1 CP play a dominant-interfering role in suppressing NMD even at substoichiometric levels relative to uncleaved UPF1? We challenged HeLa cell UPF1 function by introducing increasing amounts of plasmid DNA to express increasing but substoichiometric amounts of Δ37-UPF1-FLAG or, as a control, MYC-UPF1-FLAG WT; in parallel, we introduced empty vector DNA (θ) as an additional control ( Fig. 5a ). These transfections included the ‘Norm’ or ‘Ter’ plasmid sets. While the flexible linker and FLAG epitope of Δ37-UPF1-FLAG limit its complete resolution from endogenous UPF1 ( Fig. 5a ), the level of Δ37-UPF1-FLAG can be compared with the level of MYC-UPF1-FLAG WT in anti-FLAG blots, and since MYC-UPF1-FLAG WT is cleanly resolved from endogenous UPF1 in anti-UPF1(1–416) blots, it is possible to determine the levels of Δ37-UPF1-FLAG relative to endogenous UPF1 ( Fig. 5a ). Levels of the β-Gl Ter NMD substrate revealed that, relative to transfections employing empty vector, increasing amounts of the Δ37-UPF1-FLAG elicited an increase in the level of β-Gl Ter mRNA ( Fig. 5b ). Δ37-UPF1-FLAG expression at approximately one-third the level of endogenous UPF1 ( Fig. 5a ) yielded an ~2.4-fold higher β-Gl Ter mRNA level than in transfections employing empty vector ( Fig. 5b , red arrow). Δ37-UPF1-FLAG expression increased the level of the NMD substrate mCherry-TCRβ +JC intron mRNA ~2.3-fold ( Fig. 5c ; in the fourth sample, the decrease to ~1.5-fold and large error bars are likely due to experimental noise since the levels of β-Gl Ter mRNA continue to increase with increasing Δ37-UPF1-FLAG levels). The amount of 3 × FLAG-mCherry that derived from mCherry-TCRβ +JC intron mRNA increased with increasing yet substoichiometric amounts of Δ37-UPF1-FLAG ( Fig. 5a ). Almost no changes were observed in the level of mCherry-TCRβ +JC intron mRNA or its product protein when endogenous UPF1 was challenged with increasing but substoichiometric levels of MYC-UPF1-FLAG WT ( Fig. 5a,c ). We confirmed that the challenge of endogenous UPF1 in HEK293T cells with increasing amounts of Δ37-UPF1-FLAG, relative to empty vector control, increased β-Gl Ter mRNA levels, whereas MYC-UPF1-FLAG WT had no such effect ( Supplementary Fig. 4a,b ). 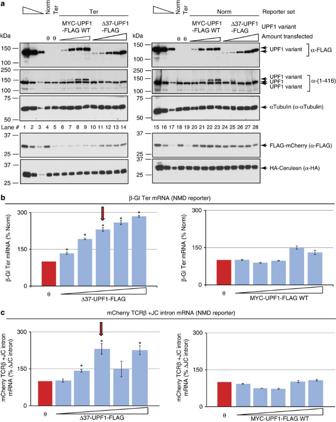Figure 5: UPF1 CP dominantly interferes with NMD at substoichiometric levels. (a) Western blots of lysates of HeLa cells transiently expressing increasing amounts of MYC-UPF1-FLAG WT or Δ37-UPF1-FLAG together with either the ‘Norm’ plasmid set (producing β-Gl Norm mRNA, 3 × FLAG-mCherry-TCRβ ΔJC intron mRNA, and MUP mRNA) or the ‘Ter’ plasmid set (producing β-Gl Ter mRNA, 3 × FLAG-mCherry-TCRβ +JC intron mRNA and MUP mRNA). Control experiments used empty vector (θ) in place of a UPF1 variant. Anti(α)-FLAG immunoblot allows unambiguous comparison of MYC-UPF1-FLAG WT and Δ37-UPF1-FLAG levels: Δ37-UPF1-FLAG exhibits ~one-third the immunoreactivity of full-length UPF1 with anti-UPF1(1–416) antiserum. Blots derive from (and are representative of) the triplicate samples analysed inb,c. (b) RT–qPCR, where the level of β-Gl Norm or Ter mRNA was first normalized to the level of MUP mRNA, and subsequently normalized to the empty-vector (θ) control (defined as 100%). The red arrow denotes the level of Δ37-UPF1-FLAG (based ona) that is comparable to the physiological level of UPF1 CP. (c) RT–qPCR, where the level of 3 × FLAG-mCherry-TCRβ ΔJC intron mRNA or 3 × FLAG-mCherry-TCRβ +JC intron mRNA was first normalized to the level of MUP mRNA, and subsequently normalized to the empty-vector (θ) control (defined as 100%). The red arrow denotes the level of Δ37-UPF1-FLAG (based ona) that is comparable to the physiological level of UPF1 CP. Error bars=s.e.m., *=P<0.05 relative to no UPF1 variant (empty vector) sample using the Student’st-test.n=3 independent biological replicates. Figure 5: UPF1 CP dominantly interferes with NMD at substoichiometric levels. ( a ) Western blots of lysates of HeLa cells transiently expressing increasing amounts of MYC-UPF1-FLAG WT or Δ37-UPF1-FLAG together with either the ‘Norm’ plasmid set (producing β-Gl Norm mRNA, 3 × FLAG-mCherry-TCRβ ΔJC intron mRNA, and MUP mRNA) or the ‘Ter’ plasmid set (producing β-Gl Ter mRNA, 3 × FLAG-mCherry-TCRβ +JC intron mRNA and MUP mRNA). Control experiments used empty vector (θ) in place of a UPF1 variant. Anti(α)-FLAG immunoblot allows unambiguous comparison of MYC-UPF1-FLAG WT and Δ37-UPF1-FLAG levels: Δ37-UPF1-FLAG exhibits ~one-third the immunoreactivity of full-length UPF1 with anti-UPF1(1–416) antiserum. Blots derive from (and are representative of) the triplicate samples analysed in b , c . ( b ) RT–qPCR, where the level of β-Gl Norm or Ter mRNA was first normalized to the level of MUP mRNA, and subsequently normalized to the empty-vector (θ) control (defined as 100%). The red arrow denotes the level of Δ37-UPF1-FLAG (based on a ) that is comparable to the physiological level of UPF1 CP. ( c ) RT–qPCR, where the level of 3 × FLAG-mCherry-TCRβ ΔJC intron mRNA or 3 × FLAG-mCherry-TCRβ +JC intron mRNA was first normalized to the level of MUP mRNA, and subsequently normalized to the empty-vector (θ) control (defined as 100%). The red arrow denotes the level of Δ37-UPF1-FLAG (based on a ) that is comparable to the physiological level of UPF1 CP. Error bars=s.e.m., *= P <0.05 relative to no UPF1 variant (empty vector) sample using the Student’s t -test. n =3 independent biological replicates. Full size image We sought to rule out the trivial explanation for the lack of Δ37-UPF1-FLAG function in NMD, that is, that the truncated protein is misfolded, by characterizing the composition of the RNP containing either MYC-UPF1-FLAG WT or Δ37-UPF1-FLAG. HEK293T cells were depleted of endogenous UPF1 using siRNA, and either MYC-UPF1-FLAG WT or Δ37-UPF1-FLAG was expressed at a level equivalent to the normal level of endogenous UPF1 ( Fig. 6 ). MYC-UPF1-FLAG WT or Δ37-UPF1-FLAG complexes were immunoprecipitated from lysates using anti-FLAG resin, each immunoprecipitate was divided in half and one half was incubated with bovine serum albumin, while the other half was incubated with RNase ONE to identify protein–protein interactions that are stabilized by RNA. 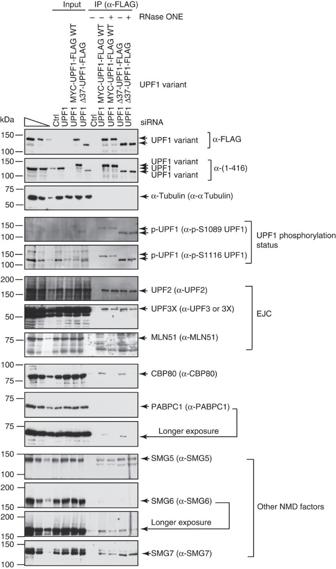Figure 6: Characterization of the UPF1 CP mRNP. Western blots of lysates of HEK293T cells transfected with either control (Ctrl) siRNA or UPF1 siRNA (100 nM) and 24 h later with plasmid encoding MYC-UPF1-FLAG WT or Δ37-UPF1-FLAG either before (Input) or after anti(α)-FLAG IP, the latter in the presence of bovine serum albumin (−) or RNase ONE (+). Representative of two independent experiments. Figure 6: Characterization of the UPF1 CP mRNP. Western blots of lysates of HEK293T cells transfected with either control (Ctrl) siRNA or UPF1 siRNA (100 nM) and 24 h later with plasmid encoding MYC-UPF1-FLAG WT or Δ37-UPF1-FLAG either before (Input) or after anti(α)-FLAG IP, the latter in the presence of bovine serum albumin (−) or RNase ONE (+). Representative of two independent experiments. Full size image Immunoblotting using antibodies directed against phosphorylated-S1089 (p-S1089) or p-S1116 in UPF1 revealed slightly enhanced phosphorylation of Δ37-UPF1-FLAG relative to MYC-UPF1-FLAG WT ( Fig. 6 ). Accumulation of C-terminal phosphates is a feature of ATPase-deficient UPF1 variants that cannot support NMD [7] , [15] , [21] , [42] . Equivalent levels of EJC components UPF2, UPF3X and MLN51, the cap-binding protein CBP80 and the poly(A)-binding protein (PABP)C1 were co-immunoprecipitated with both UPF1 variants ( Fig. 6 ). Δ37-UPF1-FLAG retrieved slightly increased levels of SMG5 and SMG7 relative to MYC-UPF1-FLAG WT in RNase-insensitive interactions ( Fig. 6 ). Equivalent levels of SMG6 were retrieved in a partially RNase-sensitive interaction ( Fig. 6 ). SMG6 association with a region outside of the UPF1 N terminus is consistent with several recent reports [7] , [52] , [53] . Our results indicate that gross misfolding of the UPF1 CP cannot explain its non-functional and dominant-interfering behaviour. We characterized the binding of MYC-UPF1-FLAG WT, Δ37-UPF1-FLAG and MYC-UPF1-FLAG D37N to PTC-containing mRNAs relative to their PTC-free counterparts by transfecting cells expressing equivalent levels of each UPF1 variant with a combination of plasmids encoding β-Gl Ter mRNA and MUP mRNA, or separately, plasmids encoding the β-Gl Norm mRNA and MUP mRNA. We measured the binding of each variant to β-Gl Ter mRNA and to its PTC-free counterpart ( Supplementary Fig. 5 ) in immunoprecipitates. As previously reported, MYC-UPF1-FLAG WT retrieved ~26-fold higher levels of the PTC-containing mRNA when adjusted for expression levels [7] and MYC-UPF1-FLAG D37N did likewise. Like the non-functional dNT UPF1 variant as well as a non-functional 4SA variant lacking four phosphorylation sites [7] , Δ37-UPF1-FLAG also retrieved β-Gl Ter mRNA relative to β-Gl Norm mRNA with an efficiency that was comparable to that of MYC-UPF1-FLAG WT and MYC-UPF1-FLAG D37N (~36-fold enrichment), despite being non-functional ( Figs 4 and 5 ). We conclude that, like the dNT variant [7] , Δ37-UPF1-FLAG is not misfolded—it can bind to the same complement of proteins as WT UPF1 and is enriched on a PTC-bearing transcript. Rather, a defect in the NMD cycle after RNA binding occurs. UPF1 cleavage upregulates genes involved in apoptosis What is the physiological relevance of UPF1 cleavage and the attenuation of NMD for cells exposed to chemotherapeutics that cause apoptosis? We interrogated the 91 genes upregulated on UPF1 downregulation in Mendell et al . [3] using the online DAVID gene ontology tool to cluster genes by function. We found a cluster (11 genes) under ‘positive regulation of programmed cell death’ ( P =2.3E−4; Supplementary Data 1 ) as well as a group of genes belonging to ‘p53 signalling pathway’ (four genes) and ‘regulation of cell cycle’ (five genes). Results from Viegas et al . [36] showed a cluster (20 genes) under ‘positive regulation of programmed cell death’ ( P =7.4E−8; Supplementary Data 1 ). DAVID analysis of results from Cho et al . [4] also yielded genes in ‘positive regulation of programmed cell death’ (10 genes) and ‘regulation of cell cycle’ (five genes). Indeed, NMD targets that we previously analysed ( Supplementary Fig. 1a ) include CDKN1A mRNA, which encodes the classical cell cycle inhibitory protein p21, and GADD45α and GADD45β mRNAs, which produce proteins involved in cell cycle arrest that also transiently upregulate CASP3 and CASP7 to promote apoptosis [54] . Thus, we hypothesized that among the transcripts upregulated on NMD attenuation is a group that the cell can exploit in response to apoptotic inducers. We generated stably transduced HeLa cell lines bearing either empty vector or a fully functional MYC-UPF1-FLAG TEV allele that harbours the tobacco etch virus (TEV) protease cleavage site substituted into the D37 position ( Fig. 4 ). Since TEV protease has no cleavage sites in the mammalian proteome [55] , transfection with a plasmid encoding two complementary MYC-tagged TEV protease fragments expressed from a bidirectional promoter allows MYC-UPF1-FLAG TEV to be specifically cleaved in living cells in the absence of apoptotic inducers ( Fig. 7a ). To identify changes in cellular mRNAs that are due UPF1 CP production, we performed RNA-Seq on the empty vector cell line and the MYC-UPF1-FLAG TEV cell line, both in the presence or absence of TEV expression, with the assumption that we would uncover direct and indirect NMD targets. 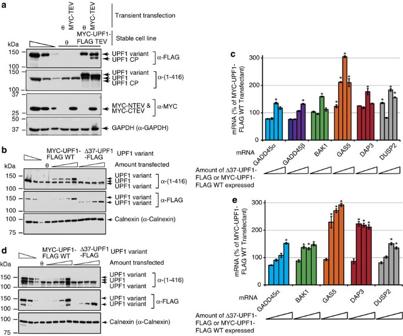Figure 7: Generation of UPF1 CP in the absence of doxorubicin upregulates genes that promote the apoptotic response to doxorubicin. (a) Western blot of lysates of HeLa cells retrovirally transduced with empty vector (θ) or the MYC-UPF1-FLAG TEV construct bearing a substitution of the TEV protease cleavage site (ENLYFQS) at D37, and subsequently transiently transfected with empty vector (θ) or a vector expressing both halves of TEV protease (each half is MYC-epitope tagged55). Both full-length MYC-UPF1-FLAG TEV and the resultant TEV-generated CP retain the C-terminal FLAG. Blots derive from (and are representative of) duplicate samples analysed by RNA-seq inSupplementary Data 2. (b) HeLa cells were transfected as inFig. 5a, but without NMD reporter sets. Blots derive from (and are representative of) the triplicate samples analysed inc. (c) RT-qPCR of mRNA from cells inbwhere the levels of the indicated transcripts in each transfectant were first normalized to the level of GAPDH mRNA, and the ratio of normalized transcript levels in the Δ37-UPF1-FLAG transfectant to the normalized transcript levels in cells expressing an equivalent amount of MYC-UPF1-FLAG WT are displayed. The normalized transcript levels in the MYC-UPF1-FLAG WT sample for each amount of transfected plasmid is set at 100%. (d) As inbbut using MCF7 cells. Blots derive from (and are representative of) the triplicate samples analysed ine. (e) As incbut using mRNA from MCF7 cells ind. Error bars=s.e.m., *=P<0.05 for Δ37-UPF1-FLAG sample relative to MYC-UPF1-FLAG WT sample using the Student’st-test.n=3 independent biological replicates. Figure 7: Generation of UPF1 CP in the absence of doxorubicin upregulates genes that promote the apoptotic response to doxorubicin. ( a ) Western blot of lysates of HeLa cells retrovirally transduced with empty vector (θ) or the MYC-UPF1-FLAG TEV construct bearing a substitution of the TEV protease cleavage site (ENLYFQS) at D37, and subsequently transiently transfected with empty vector (θ) or a vector expressing both halves of TEV protease (each half is MYC-epitope tagged [55] ). Both full-length MYC-UPF1-FLAG TEV and the resultant TEV-generated CP retain the C-terminal FLAG. Blots derive from (and are representative of) duplicate samples analysed by RNA-seq in Supplementary Data 2 . ( b ) HeLa cells were transfected as in Fig. 5a , but without NMD reporter sets. Blots derive from (and are representative of) the triplicate samples analysed in c . ( c ) RT-qPCR of mRNA from cells in b where the levels of the indicated transcripts in each transfectant were first normalized to the level of GAPDH mRNA, and the ratio of normalized transcript levels in the Δ37-UPF1-FLAG transfectant to the normalized transcript levels in cells expressing an equivalent amount of MYC-UPF1-FLAG WT are displayed. The normalized transcript levels in the MYC-UPF1-FLAG WT sample for each amount of transfected plasmid is set at 100%. ( d ) As in b but using MCF7 cells. Blots derive from (and are representative of) the triplicate samples analysed in e . ( e ) As in c but using mRNA from MCF7 cells in d . Error bars=s.e.m., *= P <0.05 for Δ37-UPF1-FLAG sample relative to MYC-UPF1-FLAG WT sample using the Student’s t -test. n =3 independent biological replicates. Full size image We note that abundance changes in either class of targets may have important effects on cellular physiology. To control for differences in the cellular responses to plasmid identity and transfection, we normalized the changes in mRNA abundance of the MYC-UPF1-FLAG TEV cell line with and without TEV protease to changes in the empty vector cell line with and without TEV protease. We recovered upregulation of mRNAs for CDKN1A (~3-fold), GADD45α (~3.7-fold) and GADD45β (4.7-fold; Supplementary Data 2 ). By expressing increasing amounts of MYC-UPF1-FLAG WT or Δ37-UPF1-FLAG in either HeLa ( Fig. 7b ) or MCF7 ( Fig. 7d ) cells and measuring the resultant changes in mRNA abundance ( Fig 7c,e ), we verified the upregulation of a subset of additional genes, each of which has individual literature-documented roles in promoting cell cycle arrest or apoptosis when its expression is increased ( Table 1 ). While we cannot explain the decrease observed for most mRNA ratios at the highest level of Δ37-UPF1-FLAG in HeLa cells (but not in MCF7 cells), we note that this expression level is greater than that observed for the CP in doxorubicin-treated cells. Table 1 NMD targets identified from RNA-seq data in Fig. 7. Full size table To support these observations, we transfected HeLa cells with substoichiometric amounts of either MYC-UPF1-FLAG WT or an equivalent amount of Δ37-UPF1-FLAG ( Supplementary Fig. 6 ), treated cells 48 h later with 5,6-dichloro-1-β- D -ribofuranosyl-1H-benzimidazole (DRB), and analysed the half-lives of endogenous NMD targets after DRB-mediated transcriptional arrest [10] . In contrast to GAPDH and β-actin mRNAs, there were noted increases in the stability of GAS5 ncRNA [56] as well as GADD45α, BAK1 and BCL3 mRNAs. Stability of ARF1 and SERPINE1 mRNAs (two Staufen-mediated mRNA decay targets) were unaffected ( Supplementary Fig. 6 ). Thus, UPF1 CP can partially attenuate NMD levels at substoichiometric amounts. Each of the genes verified from the RNA-seq data can individually promote either cell cycle arrest or apoptosis ( Table 1 ) and thus may be exploited by cells in response to chemotherapeutic treatment. Modulation of NMD activity affects doxorubicin sensitivity Two testable hypotheses follow from the observation that generating UPF1 CP in the absence of chemotherapy augments the expression of genes involved in apoptotic progression. First, inhibiting UPF1 CP production should slow the cell death response to doxorubicin. Second, inhibiting NMD through exogenous introduction of UPF1 CP or small-molecule treatment should promote doxorubicin-mediated cell death. To test the first hypothesis, we utilized HeLa cell lines stably expressing MYC-UPF1-FLAG WT or non-cleavable MYC-UPF1-FLAG D37N ( Figs 3d , 4b and 8a ), both of which support NMD. Each was expressed at ~2.7-fold above the level of endogenous UPF1 and, more importantly, at levels identical to one another ( Fig. 8a ). We exposed these cell lines to a range of doxorubicin concentrations and assessed cell viability after 16 h using an assay that detects ATP generation by living cells. At a sublethal doxorubicin concentration (0.5 μM), no statistically significant difference in viability was detected. However, as doxorubicin toxicity increased, the MYC-UPF1-FLAG D37N cell line showed increased resistance to death relative to the MYC-UPF1-FLAG WT cell line, reaching a maximum of ~2.2-fold greater survival. 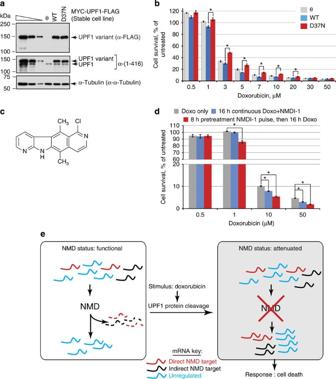Figure 8: Inhibiting UPF1 CP generation protects cells from doxorubicin challenge and inhibiting NMD promotes doxorubicin-induced cell death. (a) Western blots of HeLa cells stably expressing empty vector (θ) or equivalent amounts of MYC-UPF1-FLAG WT or MYC-UPF1-FLAG D37N. Blots derive from (and are representative of) four biological replicate samples used inb. (b) Cell lines fromawere plated in 96-well opaque tissue-culture dishes (5,000 cells per well) and exposed to the indicated concentrations of doxorubicin for 16 h. Viable cells were quantitated using a Cell Titer Glo assay. Data are normalized to untreated cells for each cell line. Errors bar=s.e.m., *=P<0.05 relative to MYC-UPF1-FLAG WT cell line samples using the Student’st-test.n=4 biological replicates. (c) Structure of NMDI-1. (d) HeLa cells were plated as inband exposed to one of three treatments 24 h later: the indicated doxorubicin concentration is provided for 16 h either alone (grey histograms) or in the presence of 10 μM NMDI-1 (blue histograms). Alternatively, cells were preincubated with 10 μM NMDI-1 for 8 h, washed three times and incubated with the indicated concentrations of doxorubicin for 16 h in the absence of NMDI-1. Viable cells were quantitated as inb. Error bars= s.e.m., *=P<0.05 relative to doxorubicin alone treatment using the Student’st-test.n=4 biological replicates. (e) Model implicating NMD modulation in establishing different cellular states (compare white box to the left and grey box to the right) by sculpting the mRNA milieu. Transcription produces mRNAs that are (red) or are not (blue) NMD targets (that is, are unregulated) or are indirect NMD targets (black). Normally, NMD is active, eliminating direct and indirect NMD targets from the mRNA milieu (left white box). However, NMD activity can be modulated by various perturbations. We show here that production of UPF1 CP(s) at substoichiometric levels downregulates NMD activity, causing direct NMD targets to enter the mRNA milieu, which secondarily causes upregulation of indirect NMD targets (right grey box). Together these changes sculpt the pool of mRNAs to one that is competent to rapidly respond to the stimulus that elicited the inhibition of NMD. Here we have shown that the stimulus (doxorubicin) attenuates NMD, facilitating an appropriate response (cell death). Figure 8: Inhibiting UPF1 CP generation protects cells from doxorubicin challenge and inhibiting NMD promotes doxorubicin-induced cell death. ( a ) Western blots of HeLa cells stably expressing empty vector (θ) or equivalent amounts of MYC-UPF1-FLAG WT or MYC-UPF1-FLAG D37N. Blots derive from (and are representative of) four biological replicate samples used in b . ( b ) Cell lines from a were plated in 96-well opaque tissue-culture dishes (5,000 cells per well) and exposed to the indicated concentrations of doxorubicin for 16 h. Viable cells were quantitated using a Cell Titer Glo assay. Data are normalized to untreated cells for each cell line. Errors bar=s.e.m., *= P <0.05 relative to MYC-UPF1-FLAG WT cell line samples using the Student’s t -test. n =4 biological replicates. ( c ) Structure of NMDI-1. ( d ) HeLa cells were plated as in b and exposed to one of three treatments 24 h later: the indicated doxorubicin concentration is provided for 16 h either alone (grey histograms) or in the presence of 10 μM NMDI-1 (blue histograms). Alternatively, cells were preincubated with 10 μM NMDI-1 for 8 h, washed three times and incubated with the indicated concentrations of doxorubicin for 16 h in the absence of NMDI-1. Viable cells were quantitated as in b . Error bars= s.e.m., *= P <0.05 relative to doxorubicin alone treatment using the Student’s t -test. n =4 biological replicates. ( e ) Model implicating NMD modulation in establishing different cellular states (compare white box to the left and grey box to the right) by sculpting the mRNA milieu. Transcription produces mRNAs that are (red) or are not (blue) NMD targets (that is, are unregulated) or are indirect NMD targets (black). Normally, NMD is active, eliminating direct and indirect NMD targets from the mRNA milieu (left white box). However, NMD activity can be modulated by various perturbations. We show here that production of UPF1 CP(s) at substoichiometric levels downregulates NMD activity, causing direct NMD targets to enter the mRNA milieu, which secondarily causes upregulation of indirect NMD targets (right grey box). Together these changes sculpt the pool of mRNAs to one that is competent to rapidly respond to the stimulus that elicited the inhibition of NMD. Here we have shown that the stimulus (doxorubicin) attenuates NMD, facilitating an appropriate response (cell death). Full size image With the first hypothesis verified, we next transiently expressed either MYC-UPF1-FLAG WT or Δ37-UPF1-FLAG in HeLa cells ( Supplementary Fig. 7a ) or MCF7 cells ( Supplementary Fig. 7c ) and challenged transfectants with doxorubicin. Although we observed statistically significant increases in sensitivity for Δ37-UPF1-FLAG transfectants relative to MYC-UPF1-FLAG WT transfectants, the effect was mild in both cell types ( Supplementary Fig. 7b,d ), likely because the toxic effects of lipofection obscure differences between the two transfected cell populations and limit the dynamic range of the assay. Therefore, we utilized a small-molecule inhibitor of NMD, NMDI-1 ( Fig. 8c ), that interferes with the interaction between UPF1 and SMG5 (refs 57 , 58 ). Application of NMDI-1 and the consequential attenuation of NMD may more fully replicate the complete inhibition of NMD mediated by the UPF1 CP generation explored here as well as UPF1 dephosphorylation and the generation of additional UPF1 CPs seen with doxorubicin ( Fig. 1c ). NMDI-1 is effective in HeLa cells, raising the levels of β-Gl Ter mRNA and another NMD target—a PTC-bearing glutathione peroxidase 1 mRNA—~3.8-fold and ~1.6-fold, respectively, at a concentration of 10 μM, which was used in subsequent experiments ( Supplementary Fig. 8a,b ). Since NMDI-1 had no effect in MCF7 cells ( Supplementary Fig. 8c,d ), we focused on HeLa cells. Because of results indicating that the efficacy of combination small-molecule treatments is affected by both drug order and timing [59] , we considered three treatment regimens. First, we challenged HeLa cells with various concentrations of doxorubicin alone. Second, we continuously co-incubated cells for 16 h with doxorubicin and NMDI-1. Third, we applied a transient pulse of NMDI-1 for 8 h, washed cells to remove NMDI-1 and then applied doxorubicin. At sublethal doses of doxorubicin (0.5 μM), none of the treatments significantly affected viability ( Fig. 8d ), in accordance with previous observations [58] . Confirming our hypothesis that inhibiting NMD should increase sensitivity to doxorubicin, continuous co-treatment with NMDI-1 led to statistically significant decreases in cell viability relative to doxorubicin treatment alone ( Fig. 8d , blue histograms). Transient pretreatment with NMDI-1 led to an even more pronounced effect and up to an ~2.5-fold reduction in cell viability at 50 μM doxorubicin relative to doxorubicin alone ( Fig. 8d , red histograms), despite the total time of exposure to NMDI-1 being half of that in the co-treatment regimen. Thus, inhibiting NMD promotes doxorubicin-mediated cell death, and conversely, inhibiting UPF1 CP generation obscures this effect. Here we observe that NMD activity is blunted during chemotherapeutic treatments (doxorubicin, staurosporine and so on) that ultimately cause apoptosis. During treatment with doxorubicin and other clinically relevant small molecules (for example, ETP), one or more UPF1 CPs are produced. The UPF1 CP that we have mapped to a region encompassing UPF1 amino acids 38–1118 acts to inhibit NMD in a dominant-interfering fashion, that is, at substoichiometric levels relative to cellular UPF1 ( Fig. 5 ; Supplementary Fig. 4 ). Inhibition is tunable—the more UPF1 CP is generated, the more PTC-containing reporter mRNA is stabilized ( Fig. 5b,c ). Increases in PTC-reporter mRNAs (~2.4-fold; Fig. 5b ) are less than those achievable using UPF1 ablation (~6–10-fold) [60] , and fold-changes in endogenous NMD targets are smaller ( Supplementary Data 1 ), indicating that substoichiometric generation of UPF1 CP may be a way to fine-tune gene expression with physiological consequences ( Fig. 8 ). The combined effects of this UPF1 CP, as well as additional UPF1 CPs ( Fig. 1c,d ), and changes to UPF1 phosphorylation status ( Fig. 1c ) all likely contribute to inhibition of NMD and upregulation of cell cycle inhibitory and apoptosis-promoting transcripts seen during doxorubicin treatment ( Figs 1a and 7 ). Small-molecule-mediated inhibition of NMD may provide an improved therapeutic strategy when delivered in combination with cytotoxic agents already in clinical use ( Fig. 8d ). Transient pretreatment with NMDI-1 before addition of doxorubicin leads to enhanced cell death relative to either doxorubicin alone or to continuous co-treatment of NMDI-1 and doxorubicin. This suggests one model for NMD involvement in enabling the establishment of different cellular states by sculpting the mRNA milieu ( Fig. 8e ). Transcription produces mRNAs that are (red) or are not (blue) NMD targets, or are indirect NMD targets (black). NMD activity degrades NMD-sensitive transcripts that are either not allowed into the pool of translated mRNAs or allowed at only low levels. Here we show that NMD activity is under the purview of the cell: NMD activity is tuned by generating a UPF1 CP ( Fig. 5 ) that inhibits NMD, allows increased amounts of NMD-sensitive transcripts into the mRNA milieu and likely also regulates indirect NMD targets. Which transcripts are direct NMD targets or indirect NMD targets may be an academic distinction to the cell. Clearly, inhibiting NMD is able to change the mRNA milieu to promote physiological consequences ( Fig. 8 ). The sum effect of these changes to the mRNA pool alters the cellular state to one that is competent to respond (via death) to the insult that elicited the inhibition of NMD (doxorubicin). Such a model explains why transient pretreatment with NMDI-1 before application of doxorubicin is a more effective treatment regimen than mere co-treatment of NMDI-1 and doxorubicin. During the pretreatment pulse, the cell has already attenuated NMD and established an mRNA milieu that can respond to doxorubicin even before doxorubicin is applied, making the response to doxorubicin (death) more rapid. An important caveat to this model is that NMD inhibition also increases the levels of truncated aberrant proteins that have detrimental effects on cellular metabolism. However, the overall response is likely the same, namely, increased sensitivity to doxorubicin. This model for NMD also extends to a recent report [13] showing that UPF1 levels are decreased by production of miR-128 in mouse embryonic NSCs. Reduction of UPF1 levels by this mechanism, and thus the inhibition of NMD, enables differentiation signals (retinoic acid) to elicit a response (neurogenesis). That many transcripts encoding proteins with diverse function are upregulated with modest magnitudes on NMD inhibition makes this an attractive way for the cell to quickly respond to diverse stimuli—only a subset of the changes made need to be exploited in response to any one stimulus. Mild upregulation of irrelevant transcripts is of little impact to cellular physiology—indeed, NMDI-1 addition has no effect at sublethal doxorubicin doses ( Fig. 8d ), mice tolerate NMDI-1 despite mild upregulation of endogenous NMD targets [57] and very recently published NMD-inhibitory compounds also show little toxicity [61] . Reagents Doxorubicin (Sigma; D1515), CHX (Sigma; C4859), ETP (Sigma; E1383), staurosporine (EMD; 569397), caspase inhibitors (EMD; set IV 80510-354), human tumour necrosis factor-α (Invitrogen; PHC3015), N -ethyl maleimide (NEM; Sigma; E3876), DRB (Sigma; D1916) and doxycycline (Sigma; D3072) were used at the concentrations and times indicated in figures and figure legends. NMDI-1 was a generous gift from David Bedwell [57] . Active recombinant Caspase 3 and 7 were from PromoKine. HeLa Tet-off cells were obtained from Clontech. Cell culture and transfections All cell lines were cultivated in DMEM (Gibco) containing 10% fetal bovine serum (Gibco) with the exception of Jurkat and Daudi cells, which were grown in RPMI-1640 (Gibco) with 10% fetal bovine serum. HeLa and MCF7 cells (ATCC) were transfected with plasmid DNA using Lipofectamine LTX (Invitrogen), and HEK293T cells were transfected with plasmid DNA using Lipofectamine 2000 (Invitrogen). Transfections using siRNA employed RNAi MAX (Invitrogen) according to the manufacturer’s directions, with the exception of Fig. 2a , which employed Oligofectamine (Invitrogen). Cells were plated in antibiotic-free medium for a minimum of 24 h before transfection and harvested 48 h after plasmid transfections or 72 h after siRNA transfections. Western blotting Cells were lysed and the protein was isolated using hypotonic buffer that consists of 10 mM Tris-Cl, pH 7.4, 10 mM NaCl, 2 mM EDTA, 0.5% Triton-X-100, 2 mM benzamidine, 1 mM PMSF, NEM (50 μg ml −1 ), 1 × phosphatase inhibitor cocktail (Roche) and 1 × protease inhibitor cocktail (Roche). After 10 min of incubation at 4 °C, NaCl was added to 150 mM, and lysates were cleared by centrifugation. Proteins were resolved using SDS–polyacrylamide gel electrophoresis, transferred to Hybond ECL nitrocellulose (GE) and probed using antibody that recognizes one of the following: UPF1(1–416) (1:2,000; ref. 8 ), p-UPF1 S1116 (1:1,000; Millipore 07–1016), p-UPF1 S1089 (1:1,000; Millipore 07–1015), Calnexin (1:2,000; Enzo Life Sciences ADISPA860), UPF2 (1:200; Santa Cruz Biotechnology C18 20227), UPF3X and 3 (1:1,000; ref. 8 ), MLN51 (1:1,000; Bethyl Laboratories A302–471), GAPDH (1:200; Santa Cruz Biotechnology 25778), CBP80 (1:1,000; Bethyl Laboratories A301–793), SMG5 (1:1,000; Abcam 33033), SMG6 (1:1,000; Abcam 57539), SMG7 (1:1,000; Bethyl Laboratories 302–170A), SMG1 (1:1,000; Cell Signaling D42D5), Cleaved Caspase 3 (1:1,000; Cell Signaling 9664), Cleaved Caspase 9 (1:1,000; Cell Signaling 7237), PARP (1:1,000; Cell Signaling 9542), Cleaved PARP (1:200; Santa Cruz Biotechnology sc56196) PLC-γ1 (1:200; Santa Cruz Biotechnology 58407), α-Tubulin (1:1,000; Cell Signaling 3873 P), FLAG (1:5,000; Sigma, clone M2 a5982), HA (1:5,000; Roche, clone 3F10 12013819001) or MYC (1:1,000; Cell Signaling, clone 9B110 2276). Immunoreactivity was assessed using SuperSignal West Pico or Femto (Pierce Biotechnology). All uncropped blots are in Supplementary Fig. 9 . siRNA sequences siRNAs used were: Control siRNA #3 (Ambion) and UPF1 siRNA (Thermo Fisher Scientific; 5′- GAUGCAGUUCCGCUCCAUUdTdT -3′). Immunoprecipitation and on-bead RNase digestion HEK293T cells were transfected as described in figure legends. Cells were lysed as described for western blotting. Input lysate protein concentrations were determined using the Bradford method (Biorad), equalized and precleared twice using protein-A conjugate agarose (Roche) for 30 min with end-over-end rotation at 4 °C. Precleared lysates were subjected to immunoprecipitation (IP) using anti-FLAG M2 Sepharose (Sigma) for 2 h at 4 °C, washed with lysis buffer supplemented to contain 0.1% Triton-X-100 and divided into two equal volumes. One-half of each IP was incubated with bovine serum albumin in RNAse ONE (Promega) reaction buffer, and the other half was incubated with 1,000 U RNAse ONE (Promega) in reaction buffer for 30 min at 4 °C. Samples were washed three times with wash buffer and eluted using 3 × FLAG peptide (Sigma) according to the manufacturer’s directions. In vitro caspase cleavage assays HEK293T cells were transfected with the indicated constructs. Cells were harvested 48 h later and anti-FLAG IP was performed as above, without RNase ONE digestion. Proteins were eluted with 3 × FLAG peptide. One microlitre of each immunoprecipitate was incubated for 5 h at 37 °C with 6 U of either Caspase 3 or Caspase 7 in caspase cleavage buffer (50 mM HEPES pH 7.2, 50 mM NaCl, 0.1% CHAPS, 10 mM EDTA, 5% glycerol and 10 mM DTT). mRNA decay assays For mRNA decay assays using actionmycin D, MCF7 cells were plated at 103,000 cells per well in 24-well dishes. After 24 h, cells either were or were not pretreated for 1 h with 5 μM doxorubicin before addition of 3 μg ml −1 actinomycin D (Sigma). Cells were harvested at the indicated time points. Doxorubicin-treated cells received doxorubucin during the chase period. For Tet-off assays, HeLa Tet-off cells (Clontech) were plated at 40,000 cells per well in 24-well dishes. After 16 h, cells were transfected with the indicated plasmids in the presence of 1 μg ml −1 doxycycline to inhibit transcription. After 48 h, cells were washed three times with medium lacking doxycycline and incubated for 5 h without doxycycline to induce transcription. Cells were then either treated with nothing, treated with 50 μM doxorubicin for 1 h before transcriptional shut-off, or treated with 50 μg ml −1 puromycin for 3 h before transcriptional shut-off. At t =0, cells were cultured in medium containing 2 μg ml −1 doxycycline to induce shut-off and subsequently harvested at the indicated time points. For cells treated with doxorubicin or puromycin, these compounds were included in the chase. RT–qPCR was used to assess mRNA levels during the chase time. Data for actinomycin D decay assays ( Fig. 1a ) as well as for Tet-off decay assays ( Fig. 1b ), with the exception of the no-treatment β-Gl 39 Ter mRNA data, were fitted to best-fit linear regression lines because they clearly exhibited single component decay kinetics. In contrast, the no-treatment β-Gl 39 Ter mRNA has been shown to decay with two-component kinetics [62] . For DRB-treated mRNA decay assays, HeLa cells were transfected with the indicated plasmids using Lipofectamine LTX. After 48 h, cells were treated with 100 μg ml −1 DRB (Sigma). Cells were harvested at the indicated time points and RT–qPCR was used to assess transcript levels. TEV cleavage and RNA-seq For the TEV cleavage experiments, stably transduced HeLa cell lines were plated at 200,000 cells per well in a six-well dish and cultured without antibiotics for 48 h. Either the bidirectional TEV protease-encoding plasmid or empty vector was introduced, and cells were harvested and flash frozen 16 h later. RNA was processed as for RT–qPCR. Biological duplicates of each sample (each duplicate consisted of six pooled wells) were used for sequencing. Total-cell RNA was submitted to the Whitehead Institute Genome Technology Core for RNA-seq. RNA concentrations were determined using a NanopDrop 1000 spectrophotometer (NanoDrop, Wilmington, DE) and RNA quality was assessed using an Agilent Bioanalyzer (Agilent, Santa Clara, CA). Poly(A) + libraries were prepared using the automated IntegenX Apollo system. Sequencing was performed using an Illumina HiSeq 2500 in 40-bp single-read mode. Data analysis was performed by the University of Rochester Genomics Research Center. Raw reads generated from the Illumina HiSeq2500 sequencer were demultiplexed using configurebcl2fastq.pl version 1.8.3. Low-complexity reads and vector contamination were removed using sequence cleaner (‘seqclean’) and the NCBI univec database, respectively. The FASTX toolkit (fastq_quality_trimmer) was applied to remove bases with quality scores below Q =13 from the end of each read. Processed reads were then mapped to the UCSC Hg19 genome build using SHRiMP version 2.2.3, and differential expression analysis was performed using Cufflinks version 2.0.2; specifically, cuffdiff2 and usage of the general transfer format annotation file for the given reference genome. Pooled duplicate values were used for analyses. Specifically, fold-change in Fragments Per Kilobase of transcript per Million (FPKM) values for cell lines stably transduced with empty vector and subsequently transiently transfected with TEV-encoding plasmid or empty vector were calculated. The same calculation was performed with FPKM values for the MYC-UPF1-FLAG TEV cell line. These values obtained for the MYC-UPF1-FLAG TEV cell line were then normalized to the fold-change value obtained for the empty vector stable cell line, and this calculation was performed for all genes represented. Cell survival assays Cells were plated in white opaque 96-well plates using multichannel pipettors for accuracy and treated as described in the figure legends. CellTiter-Glo luminescent assays (Promega) were performed according to the manufacturer’s directions. Data were collected using a SpectraMax M2 plate reader. Accession codes: All sequencing data have been deposited at www.ncbi.nlm.nih.gov/sra (accession SRP044296 ). How to cite this article: Popp, M. W. and Maquat, L. E. et al . Attenuation of nonsense-mediated mRNA decay facilitates the response to chemotherapeutics. Nat. Commun. 6:6632 doi: 10.1038/ncomms7632 (2015).